Ruthenium(II)-catalysed remote C–H alkylations as a versatile platform tometa-decorated arenes The full control of positional selectivity is of prime importance in C–H activation technology. Chelation assistance served as the stimulus for the development of a plethora of ortho -selective arene functionalizations. In sharp contrast, meta -selective C–H functionalizations continue to be scarce, with all ruthenium-catalysed transformations currently requiring difficult to remove or modify nitrogen-containing heterocycles. Herein, we describe a unifying concept to access a wealth of meta -decorated arenes by a unique arene ligand effect in proximity-induced ruthenium(II) C–H activation catalysis. The transformative nature of our strategy is mirrored by providing a step-economical entry to a range of meta -substituted arenes, including ketones, acids, amines and phenols—key structural motifs in crop protection, material sciences, medicinal chemistry and pharmaceutical industries. The functionalization of otherwise inert C–H bonds by means of transition metal catalysis has emerged as an increasingly powerful platform in organic synthesis, with transformative applications to medicinal chemistry, material sciences and drug design [1] , [2] , [3] , [4] , [5] , [6] , [7] , [8] , [9] , [10] . Since the substrates of interest display a variety of C–H bonds with close dissociation energies, achieving positional selectivity in intermolecular C–H transformations is paramount [11] , [12] , [13] , [14] , [15] . Thus, chelation assistance has proven particularly instrumental for proximity-induced ortho -C–H functionalizations [16] , [17] , [18] , [19] . In stark contrast, remote arene functionalizations continue to be challenging, with major recent progress being achieved by inter alia complementary palladium [20] , [21] , [22] , [23] , [24] , [25] , [26] , [27] , [28] , [29] , iridium [30] , [31] , rhodium [32] and ruthenium [33] , [34] , [35] , [36] , [37] , [38] , [39] catalysis through steric control, template assistance, weak hydrogen bonding, transient mediators or catalytic σ-activation by ortho -C–H metalation ( Fig. 1a ) [40] . Despite undisputable advances, these methods typically offer access to only a single compound class. Furthermore, all protocols for ruthenium-catalysed meta -C–H functionalization [33] , [34] , [35] , [36] , [37] , [38] , [39] continue to be restricted to nitrogen-containing heterocycles, such as 2-arylpyridines, as the directing group. Since such heteroarenes are difficult to modify or remove [39] , [41] , the synthetic utility of this strategy is significantly compromised. Within our program on sustainable C–H activation, we have now addressed these major limitations in C–H activation technology by developing remote imine C–H functionalizations by a unique arene ligand effect, unleashing the full potential of C–H activation technology. Our approach is characterized by an expedient substrate scope, providing a broad access to various meta -decorated arenes, including synthetically meaningful ketones, alcohols, amines and acids, that constitute integral structural motifs in material sciences, crop protection and drug design ( Fig. 1b ) [42] , [43] . Notable features of our findings are not limited to (1) a remarkable arene ligand effect in ruthenium C–H activation chemistry, (2) a distinct catalyst design and (3) a tandem multicatalysis [44] approach involving both remote meta - and ortho -C–H functionalization with the aid of a single ruthenium(II) catalyst manifold. 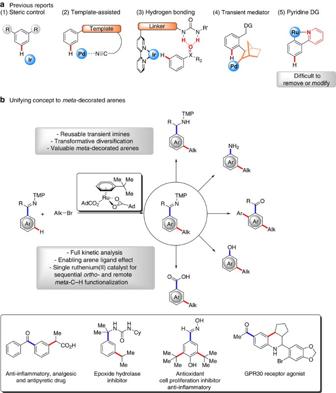Figure 1: Transformative ruthenium(II)-catalysedmeta-C–H functionalization regime. (a) Previous reports: selectivity control by (1) steric interactions, (2) template auxiliaries, (3) hydrogen bonding, (4) transient mediator and (5) difficult to remove or modify pyridines. (b) Unifying concept to a wealth ofmeta-decorated arenes. Figure 1: Transformative ruthenium(II)-catalysed meta -C–H functionalization regime. ( a ) Previous reports: selectivity control by (1) steric interactions, (2) template auxiliaries, (3) hydrogen bonding, (4) transient mediator and (5) difficult to remove or modify pyridines. ( b ) Unifying concept to a wealth of meta -decorated arenes. Full size image Development of meta -C–H alkylation We commenced our studies by probing the effect exerted by carboxylates and solvents on the challenging meta -C–H alkylation of synthetically useful ketimines 1 ( Table 1 and Supplementary Table 1 ). Sterically congested 1-AdCO 2 H ( 4 ) [45] was found to be an efficient ligand for the desired remote C–H functionalization process (entries 1 and 2). Notably, among a variety of solvents, tert -butylbenzene set the stage for a particularly effective meta -C–H functionalization catalysis that strongly contrasts to the previously employed 1,4-dioxane and toluene solvents (entries 1–5). Given the power of mono-protected amino acids (MPAAs) in C–H activation [35] , [46] , [47] , we also explored different MPAAs in the meta -C–H functionalization process (entries 6–9), with Piv-Ile-OH ( 5 ) emerging as the best in class (entries 9–11). Table 1 Reaction development for meta -selective C–H functionalization. Full size table Substrate scope The versatility of the optimized ruthenium(II)-catalysed meta -C–H alkylation was explored with substituted ketimines 1 and tertiary bromides 2 , initially employing the ruthenium(II) catalyst derived from the MPAA Piv-Ile-OH ( 5 ). The catalytic system was found to be versatile, yet the ruthenium(II) biscarboxylate catalyst generally proved more powerful ( Fig. 2 ). We were pleased to observe that both tertiary and secondary alkyl bromides 2 were compatible electrophiles in the carboxylate-assisted ruthenium(II)-catalysed meta -C–H functionalization. A range of electronically differentiated ketimines 1 performed well under the optimized reaction conditions with both cyclic and acyclic tertiary alkyl bromides 2 . It is noteworthy that the alkyl bromide 2e containing a highly reactive alkyl chloride motif furnished the desired product 3ae with excellent levels of chemoselectivity. The remarkable versatility of the optimized ruthenium catalyst was reflected by fully tolerating synthetically valuable functional groups, such as chlorides, heteroarenes, ester, ketones, thioethers or amines, within intramolecular as well as intermolecular competition experiments, including a robustness screen [48] protocol (see the Supplementary Table 3 ). 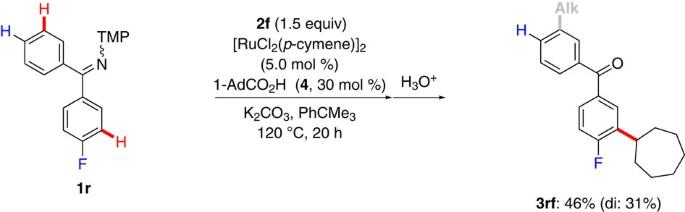Figure 3: Intramolecular competition experiment. Alkylation occurs on the more electron-deficient aromatic group. Propiophenone-derived ketimine 1e - f underwent the meta -cycloheptylation to selectively deliver the desired products 3 , while an aldimine substrate gave thus far only less satisfactory yields of 20%. Likewise, the naphthalene derivative 1l furnished meta -substituted arene 3lf – 3lm as the sole products by positional selective C–H functionalization, while the structurally complex steroid 3of could be prepared by remote C–H activation. It is noteworthy that the corresponding 3,4,5-trimethoxyphenyl (TMP)-amine could be recovered after its traceless removal in high yields (see 3eb ). 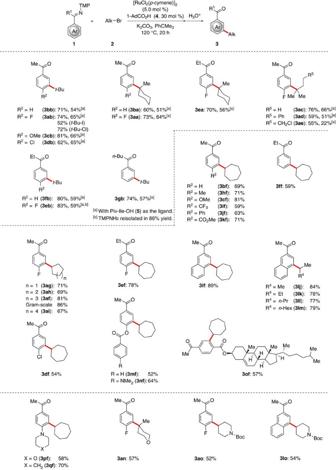Moreover, synthetically useful Lewis-basic heterocycles, such as morpholine, pyran and piperidine, were fully accepted by the robust ruthenium(II) catalysis regime. Figure 2: Substrate scope. Versatility of the ruthenium(II)-catalysedmeta-alkylation. Figure 2: Substrate scope. Versatility of the ruthenium(II)-catalysed meta -alkylation. Full size image Mechanistic considerations Given the unique efficacy of the ketimine-assisted meta -C–H functionalization by ruthenium(II) catalysis, along with the unconventional solvent effect, we became attracted to delineating its mode of action. To this end, intra- and intermolecular competition experiments revealed the meta -C–H alkylation to exclusively occur on the more electron-deficient aromatic moieties ( Fig. 3 , and the Supplementary Figs 1 and 2 ), with the geometric isomers of substrate 1r undergoing facile interconversion even at ambient temperature ( Supplementary Fig. 3 ). It is noteworthy that these observations strongly contrast with the trend previously observed in meta -sulfonylations [38] and alkylations [37] of 2-phenylpyridines, in which electron-rich arenes usually reacted preferentially. In contrast to previous proposals [38] , [49] , our findings thus render an electrophilic substitution manifold unlikely to be operative here. Figure 3: Intramolecular competition experiment. Alkylation occurs on the more electron-deficient aromatic group. Full size image Furthermore, the use of typical radical scavengers ( Fig. 4a ), enantiomerically enriched substrate 2m ( Fig. 4b ) and the diastereomerically pure alkyl halides 2p provided strong support for a radical-based mechanism ( Fig. 4c ). 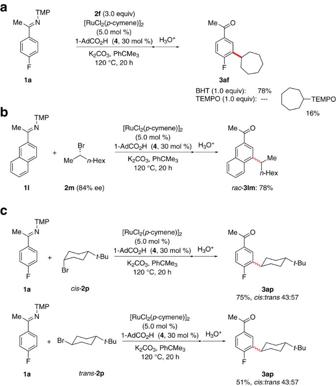Figure 4: Mechanistic studies. Probing a radical-based mechanism by (a) the addition of radical scavengers (b) the use of enantiomerically enriched alkyl halide2mand (c) the use of diasteromerically pure2p. Figure 4: Mechanistic studies. Probing a radical-based mechanism by ( a ) the addition of radical scavengers ( b ) the use of enantiomerically enriched alkyl halide 2m and ( c ) the use of diasteromerically pure 2p . Full size image Detailed kinetic experiments with mono-metallic catalyst [Ru(O 2 CAd) 2 ( p -cymene)] ( 6 ) highlighted a first-order dependence with respect to both the single-component catalyst 6 and the ketimine 1a ( Fig. 5 ), with saturation kinetics being observed for the alkyl bromide 2a (see the Supplementary Fig. 4 ). An Arrhenius plot analysis highlighted an activation barrier of 99 kJ mol −1 . To rationalize the unique effect exerted by the aromatic solvent tert -butylbenzene, we independently prepared the novel single-component complex 7 . It is noteworthy that the well-defined catalyst 7 featured a significantly reduced induction period, along with an overall improved robustness and catalytic efficacy, indicating a unique arene ligand effect in ruthenium-catalysed C–H activation catalysis. 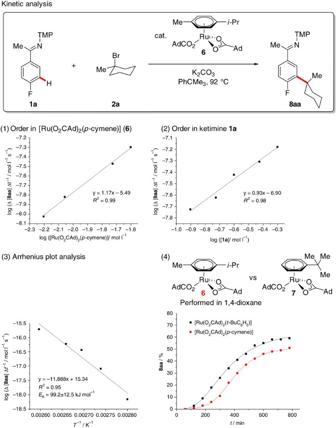Figure 5: Kinetic analysis. Order in (1) catalyst6and (2) reagent1a, for detailed information, see theSupplementary Information. (3) Arrhenius plot analysis. (4) Comparison of performance with single-component ruthenium(II) arene catalysts6and7. Figure 5: Kinetic analysis. Order in (1) catalyst 6 and (2) reagent 1a , for detailed information, see the Supplementary Information . (3) Arrhenius plot analysis. (4) Comparison of performance with single-component ruthenium(II) arene catalysts 6 and 7 . Full size image Late-stage diversification The outstanding synthetic utility of the remote [50] imine C–H functionalization approach for late-stage diversification of the thus obtained meta -alkylated arenes was reflected by operationally simple transformations in a user-friendly one-pot fashion ( Fig. 6 ). Facile reduction of the ketimines 8 , hence, provided valuable benzyl amine derivatives 9 . Gratifyingly, sequential meta -C–H alkylation followed by ortho -C–H arylation or alkylation provided access to densely substituted aromatics 10 with no additional catalyst being required, showcasing the enabling power of our approach within a user-friendly multicatalysis regime. The unique synthetic versatility of the meta -substituted arenes 3 was further illustrated by transformative diversifications ( Fig. 6 ), forming useful building blocks and biologically significant motifs, such as carboxylic acids 11 , and indoles 12 . In this regard, the preparation of meta -substituted phenols 13 and anilines 14 is particularly noteworthy, since classical methods of organic synthesis, such as the Friedel–Crafts reactions, fall short in providing access to the meta -decorated scaffolds due to the substrate’s inherent bias for ortho / para -guided selectivity. 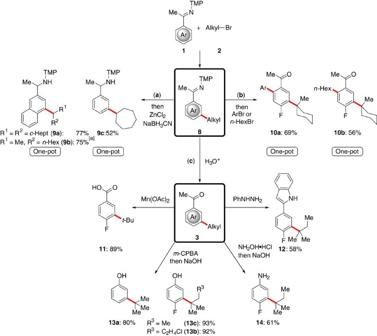Figure 6: Late-stage diversification. Themeta-C–H functionalization of ketimines1as transformative platform into synthetically meaningful and biologically significant compounds. For detailed information, see theSupplementary Information. (a) One-pot remote-C–H functionalization/reduction.[a]dr=1.0:1.2. (b) One-potmeta-C–H alkylation andortho-C–H arylation/alkylation regime. (c) Late-stage diversification to access acids11, indoles12, phenols13and anilines14. Ar=4-MeOC6H4. Figure 6: Late-stage diversification. The meta -C–H functionalization of ketimines 1 as transformative platform into synthetically meaningful and biologically significant compounds. For detailed information, see the Supplementary Information . ( a ) One-pot remote-C–H functionalization/reduction. [a] dr =1.0:1.2. ( b ) One-pot meta -C–H alkylation and ortho -C–H arylation/alkylation regime. ( c ) Late-stage diversification to access acids 11 , indoles 12 , phenols 13 and anilines 14 . Ar=4-MeOC 6 H 4 . Full size image In summary, we have presented a versatile concept for the step-economical preparation of meta -substituted arenes by remote C–H functionalization. Henceforth, a considerable arene ligand effect set the stage for a powerful ruthenium(II) catalysis manifold that expedited efficient secondary and tertiary C–H alkylations of easily accessible ketimines with exceptional positional selectivity. Operationally simple one-pot protocols delivered synthetically useful meta -functionalized benzyl amines, while multicatalytic C–H functionalizations produced densely meta -/ ortho -substituted arenes within a one-pot process. The transformative nature of the approach was highlighted by the preparation of a wealth of meta -substituted arenes, including ketones, amines, indoles, acids and phenols. General techniques Catalytic reactions were performed under a N 2 atmosphere using pre-dried glassware and standard Schlenk techniques. 1,4-Dioxane was dried over sodium and freshly distilled under N 2 . Yields refer to isolated compounds, estimated to be >95% pure as determined by 1 H-nuclear magnetic resonance ( 1 H-NMR) and gas chromatography. Thin-layer chromatography was performed on Merck, TLC Silica Gel 60 F 254 with detection under ultraviolet light at 254 nm. Chromatographic separations were carried out on Merck Geduran SI-60 (0.040–0.063 mm, 230–400 mesh ASTM). Infrared spectra were recorded on a Bruker FT-IR alpha-P device. Electron ionization mass spectrometry was recorded on Jeol AccuTOF at 70 eV; electrospray ionization mass spectrometry was recorded on Bruker Daltonik micrOTOF and maXis and LIFDI with a Linden CMS. Elemental analyses were measured on an Elementar Vario EL 3 analyser. Melting points were measured on Stuart melting point apparatus SMP3; values are uncorrected. NMR spectroscopy was performed at 300, 400 or 500 MHz ( 1 H-NMR), 75, 100 or 125 MHz ( 13 C-NMR, APT), 282, 376 or 470 MHz ( 19 F-NMR) and 282 or 376 MHz ( 19 F{ 1 H}) on Bruker Avance III HD 300, Avance III 300, Avance III 400, Avance III HD 500, Varian Unity-300, Inova 500 and Inova 600 instruments. If not otherwise specified, chemical shifts ( δ ) are provided in p.p.m. and spectra referred to non-deuterated solvent signal. Analytical high-performance liquid chromatography analysis was performed on Agilent 1260 Infinity equipped with Daicel CHIRALPAK IC-3 (4.6 mm × 250 mm, 3 μm particle size, 1 ml min −1 flow rate). Optical rotary power was measured on Jasco P-2000 polarimeter as a 0.04 g per 100 ml solution in MeOH at 589 nm and 23.0 °C. For NMR spectra of all products in this article, see the Supplementary Figs 5–60 . General procedure for catalysed meta -C–H alkylation Ketimine 1 (0.50 mmol) [RuCl 2 ( p -cymene)] 2 (15.3 mg, 25.0 μmol), 1-AdCO 2 H (27.3 mg, 0.15 mmol) and K 2 CO 3 (138 mg, 1.00 mmol) were placed in a pre-dried 25 ml pressure tube. The reaction tube was then evacuated and backfilled with nitrogen three times. Alkyl bromide 2 (1.50 mmol) and PhCMe 3 (2.0 ml) were added and the mixture was stirred at 120 °C for 20 h. At ambient temperature, HCl (2 N, 3.0 ml) was added, and the resulting mixture was stirred for an additional 3 h, and extracted at ambient temperature with EtOAc or Et 2 O (3 × 20 ml). The combined organic layers were dried over Na 2 SO 4 and concentrated in vacuo . Purification of the residue by column chromatography ( n -hexane/EtOAc or n- pentane/Et 2 O) yielded phenone 3 . Data availability The authors declare that the data supporting the findings of this study are available within the article and its Supplementary Information files. All data are also available from the authors on reasonable request. How to cite this article: Li, J. et al . Ruthenium(II)-catalysed remote C–H alkylations as a versatile platform to meta -decorated arenes. Nat. Commun. 8, 15430 doi: 10.1038/ncomms15430 (2017). Publisher’s note : Springer Nature remains neutral with regard to jurisdictional claims in published maps and institutional affiliations.